Responsive nematic gels from the self-assembly of aqueous nanofibres Aqueous nanofibres constructed by the self-assembly of small amphiphilic molecules can become entangled to form hydrogels that have a variety of applications including tissue engineering, and controlled drug delivery. The hydrogels are formed through the random physical cross-linkings of flexible nanofibres. Here we report that self-assembled nanofibres with a nematic substructure are aligned into a nematic liquid crystal and are spontaneously fixed in the aligned state to give rise to anisotropic gels. The liquid-crystal gels respond to temperature by transforming into a fluid solution upon cooling. Thus, the nanofibre solution can be mixed with cells at room temperature and then can be transformed into gels to encapsulate the cells in a three-dimensional environment upon being heated to physiological temperatures. We found that the cells grow within the three-dimensional networks without compromising the cell viability, and that subsequent cooling triggers the encapsulated cells to be released through a sol–gel transition. Molecular self-assembly into one-dimensional (1D) objects has been the subject of intense study as a means of creating intelligent materials and devices for nanotechnology [1] , [2] , [3] , [4] . One of the most ubiquitous 1D self-assemblies in nature is that of cytoskeleton components such as actin filaments and microtubules, which are responsible for resisting tension and maintaining the cellular shape. The self-assembled nanofibres in aqueous solution become easily entangled with one another to form networks that are well-suited as scaffolds for the gelation of solvent molecules and three-dimensional (3D) cell culture [5] , [6] , [7] , [8] , [9] , [10] . In contrast to polymer networks, these supramolecular gels can be easily disintegrated by changing their environments because their formation is completely reversible. The dynamic nature of the aggregates allows them to adapt to the changes in their surroundings. This adaptation has a crucial role in the artificial extracellular matrix that mimics the in vivo cell- and tissue-growth situation [11] , [12] , [13] , [14] . Another interesting aspect regarding the artificial network structures is the possibility of implementing rapid responses to external triggers. The combination of the principles of 3D networks with responsive properties has generated a new class of intelligent nanomaterials that can be used as functional biomaterials and in controlled drug delivery systems [15] , [16] , [17] , [18] , [19] , [20] . Small amphiphilic molecules, based on responsive building blocks, have been shown to be useful molecular modules for the creation and stabilization of responsive hydrogels based on non-covalent interactions [21] , [22] , [23] , [24] . Typical examples include peptide amphiphiles based on elastin-like oligopeptides, poly( N -isopropyl acrylamide) and poly(ethylene oxide) chains that form nanofibres and, subsequently, entangle with one another to form stimuli-responsive hydrogels [25] , [26] . The introduction of such responsive segments into self-assembling block molecules not only enhances their solubility in aqueous solvents but also endows the nanofibres with a responsive property as a result of thermally regulated dehydration [27] . Although numerous examples of stimuli-responsive gels have been reported, most of them are based on isotropic networks [28] , [29] . Herein we report the formation in aqueous solution of supramolecular nanofibres, with a nematic substructure, that are aligned parallel to each other to form nematic networks ( Fig. 1 ). Unlike conventional gels, the anisotropic opaque gel reversibly transforms into a transparent solution upon cooling. Thus, the nanofibre solution can be mixed with cells at room temperature and transformed into gels to encapsulate the cells in a 3D environment when the solution is heated to physiological temperatures. We found that the cells grow within the 3D gels and that subsequent cooling triggers the cells to be released from the gels into the solution. 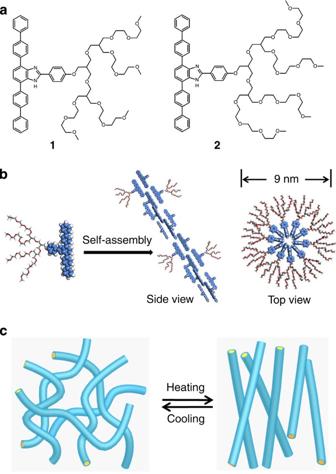Figure 1: Molecular structure and self-assembly. (a) Molecular structure of laterally grafted rod amphiphiles. (b) Schematic representation of the molecular packing arrangements of the nanofibres. (c) Schematic representation of a reversible isotropic sol–nematic gel phase transition of supramolecular nanofibres. Figure 1: Molecular structure and self-assembly. ( a ) Molecular structure of laterally grafted rod amphiphiles. ( b ) Schematic representation of the molecular packing arrangements of the nanofibres. ( c ) Schematic representation of a reversible isotropic sol–nematic gel phase transition of supramolecular nanofibres. Full size image Molecular synthesis and self-assembly The responsive gel is derived from the self-assembly of laterally grafted rod amphiphiles that consist of a penta- p -phenylene rod and a laterally grafted dendritic oligoether chain through an imidazole linkage [30] , [31] (see Supplementary Methods and Supplementary Fig. S1 ). The aggregation behaviour of the molecules was investigated in aqueous solution using transmission electron microscopy (TEM). Molecule 1 , which is based on a shorter di(ethylene oxide) chain, was insoluble in water; however, the addition of MeOH induces self-assembly of the nanostructures. 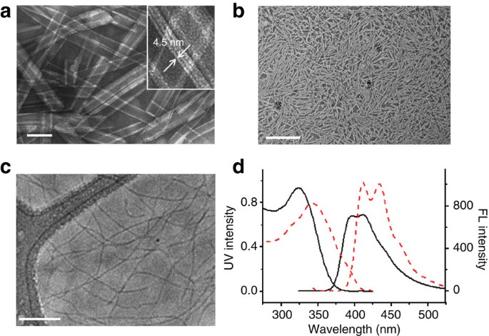Figure 2: Transmission electron microscopy (TEM) images and optical characterizations. (a) TEM image of1from a 0.1 wt% mixed solution (H2O:MeOH=7:3 v/v). The inset is the high-magnification image. (b) TEM image of2from a 0.05 wt% aqueous solution (stained with uranyl acetate). (c) Cryo-TEM image of a 0.05 wt% aqueous solution of2. (d) Absorption and emission spectra of 0.01 wt% of2in CHCl3(black and solid line) and in aqueous solution (red and dashed line). The scale bars ina–care 100, 200 and 100 nm, respectively. FL, fluorescence; UV, ultraviolet. Figure 2a shows a micrograph obtained from a 0.01 wt% mixed solution (H 2 O:MeOH=7:3 v/v) of 1 cast onto a TEM grid. The TEM image of the sample, which was negatively stained with uranyl acetate, shows the formation of tubules with single- or multiwalled structures. The appearance of the nanotubes consists of a white periphery separated by a dark interior, which is characteristic of projection images of hollow tubules. The walls consist of multilayers with a primary spacing of ~4.5 nm. Given the laterally extended molecular length (2.3 nm by the Corey–Pauling–Koltun molecular model), the 4.5 nm width is approximately twice the laterally extended molecular length. This result suggests that the rod segments within the domains are parallel to the layer planes and that the rod segments are aligned parallel to each other to form an in-plane nematic-like organization. Similar to the bulk organization of other laterally grafted rod-coil molecules [30] , [31] ( Supplementary Fig. S2 ), the tubules seem to stem from the rolling-up of the initially formed anisotropic layers along the rod direction. Figure 2: Transmission electron microscopy (TEM) images and optical characterizations. ( a ) TEM image of 1 from a 0.1 wt% mixed solution (H 2 O:MeOH=7:3 v/v). The inset is the high-magnification image. ( b ) TEM image of 2 from a 0.05 wt% aqueous solution (stained with uranyl acetate). ( c ) Cryo-TEM image of a 0.05 wt% aqueous solution of 2 . ( d ) Absorption and emission spectra of 0.01 wt% of 2 in CHCl 3 (black and solid line) and in aqueous solution (red and dashed line). The scale bars in a – c are 100, 200 and 100 nm, respectively. FL, fluorescence; UV, ultraviolet. Full size image We envisioned that an increment of the volume fraction of the dendritic flexible chain would enforce the layers to split along the rod direction into elongated fibres to reduce steric crowdings between the larger dendritic chains [32] . Indeed, the TEM image of 2 , which is based on a longer tri(ethylene oxide) chain that was obtained from a 0.01 wt% aqueous solution, shows the formation of nanofibres with a uniform diameter of ~9 nm and lengths of several micrometres ( Fig. 2b ). As a further analysis, small-angle X-ray scattering experiments were performed on highly concentrated solutions. The small-angle X-ray scattering pattern of a 30-wt% aqueous solution of 2 displayed three broad reflections with the ratio of 1:√2:2 in the low-angle region; the reflections were assigned to a 2D tetragonal columnar structure with a lattice constant of 9.4 nm, which is close to the value obtained from TEM images ( Supplementary Fig. S4b ). This diameter dimension, which exhibits a large discrepancy when compared with the molecular dimensions (~5.5 nm), suggests that the rod segments are directed parallel to the fibre axis within the aromatic core that is surrounded by hydrophilic dendritic chains. The formation of the elongated objects in the bulk solution was further confirmed by dynamic light scattering experiments in which the angular dependence of the apparent diffusion coefficient ( D app ) is consistent with the value predicted for cylindrical aggregates ( Supplementary Figs S3 and S4 ). To gain insight into the packing arrangements of the rod segments within the 1D aromatic domains, we performed ultraviolet–visible and fluorescence measurements on the aqueous solution (0.01 wt%) of 2 ( Fig. 2d ). The absorption spectrum of the aqueous solution shows a broad transition with a maximum of 350 nm that is red-shifted relative to that observed in CHCl 3 solution. Notably, the fluorescence spectrum of the aqueous solution shows an enhanced strong emission compared with the CHCl 3 solution. Both the red-shifted absorption and the enhanced fluorescence intensity are characteristic of J-type aggregates of chromophores, which suggests that the rod segments are aligned with a nematic-like slipped arrangement within the 1D aromatic domains [33] , [34] . On the basis of this result, together with the diameter of the fibre, the rod segments are considered to be aligned parallel to each other along the fibre axis, thereby giving rise to highly fluorescent nanofibres ( Fig. 1b ). This result is in significant contrast to conventional nanofibres based on conjugated rods that show strong fluorescence quenching [1] , and implies how to construct fluorescent 1D nanostructures without quenching. Thermo-responsive properties of supramolecular nanofibres The formation of nanofibres with an oligoether dendritic exterior suggests that the aqueous solution would exhibit thermo-responsive behaviour because the degree of hydration of the ethylene oxide chains decreases with increasing temperature. 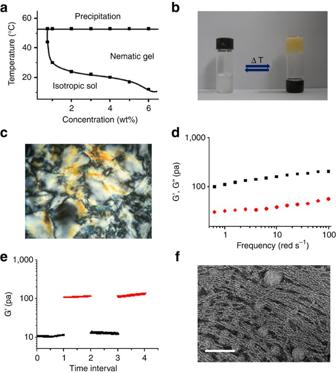Figure 3: Sol–gel interconversion. (a) Phase diagram plotted in terms of the concentration of2versus temperature. (b) Optical image of the reversible transformation from the aqueous solution to the nematic gel. (c) A representative optical polarized micrograph of a nematic gel phase. (d)G′ (black square) andG″ (red circle) values of the nematic gels of2(3 wt% aqueous solution) on frequency sweep (from 0.1 to 100 rad s−1). (e) Temperature-dependence of the storage modulus (G′) for a 3 wt% aqueous preparation of2(data were collected at 10 °C (black) and 30 °C (red) for 20 min time intervals). (f) TEM image of a 1 wt% nematic gel of2at 30 °C. Scale bar, 100 nm. As shown in Figure 3a , the transparent nanofibre solutions at concentrations greater than 0.8 wt% undergo turbid gelation upon heating and the resulting gels appear to be strongly birefringent. This appearance of birefringence is indicative of a transition between two states with different alignments of the nanofibres. The optical polarized micrograph of the gels shows a thread-like texture ( Fig. 3c ), that is, characteristic of a nematic liquid crystalline phase that rapidly transforms into an isotropic liquid upon cooling. The transition temperature decreases to 10 °C as the concentration is increased up to 6.0 wt%. As shown in Figure 3d , the dynamic viscoelasticity measurements of an aqueous solution (3 wt%) show a frequency-independent storage modulus ( G ′), the value of which is much larger than that of the loss modulus ( G ″). This result indicates the formation of a nematic gel at temperatures above the transition temperature [35] . The storage modulus measurements as a function of temperature for the heating/cooling cycles indicate that the sol–gel transition is completely reversible with subsequent temperature cycles ( Fig. 3e ). At 30 °C, the solution exists as a self-supporting gel ( G ′=120 Pa). When the solution is cooled to 10 °C, gel dissolution and low G ′ values are observed, which is consistent with a freely fluid solution that immediately recovers to the gel state upon subsequent heating. Figure 3: Sol–gel interconversion. ( a ) Phase diagram plotted in terms of the concentration of 2 versus temperature. ( b ) Optical image of the reversible transformation from the aqueous solution to the nematic gel. ( c ) A representative optical polarized micrograph of a nematic gel phase. ( d ) G ′ (black square) and G ″ (red circle) values of the nematic gels of 2 (3 wt% aqueous solution) on frequency sweep (from 0.1 to 100 rad s −1 ). ( e ) Temperature-dependence of the storage modulus ( G ′) for a 3 wt% aqueous preparation of 2 (data were collected at 10 °C (black) and 30 °C (red) for 20 min time intervals). ( f ) TEM image of a 1 wt% nematic gel of 2 at 30 °C. Scale bar, 100 nm. Full size image The TEM image of the gel after it was dried on a carbon-coated copper grid reveals parallel alignments of the nanofibres at higher temperatures ( Fig. 3f ). These parallel alignments demonstrate that the gel formation is attributable to the nematic alignments of the randomly oriented nanofibres. Consequently, heating the solution drives the fluid state to transform into anisotropic gels in which the elementary fibres are interconnected with each other to immobilize solvent molecules. This thermo-responsive solution behaviour can be explained by considering the entropically driven dehydration of the oligoether chains, as the solution is heated [36] . This dehydration allows the exterior of the nanofibres to become more hydrophobic, thus resulting in enhanced hydrophobic interactions between adjacent nanofibres to form gels. Also, the lyotropic liquid crystal forms at an unususally low concentration (0.8 wt%) of the rod segment. This unusual solution behaviour seems to stem from the formation of the supramolecular nanofibres with a high persistent length that is imparted by a nematic substructure of the rod segments aligned along the fibre axis. Encapsulation and release of live cells The spontaneous fixation of the nanofibres in the gel state under physiological conditions holds great promise for the formation of artificial 3D cell culture scaffolds that mimic the natural extracellular matrix [13] , [37] . In particular, the stiffness of the gels (120 Pa in storage modulus) is suitable to maintain mammalian cells in 3D environments for tissue regeneration applications [38] . As the first step towards this direction, we prepared C2C12 (myoblast, mouse muscle adherent cells) cell-containing gels for a 3D cell culture. After mixing C2C12 cells with the nanofibre solutions, the solution was heated to the gelation temperature to encapsulate the cells within the gel matrix ( Fig. 4a,b ). These adherent cells remains alive for at least 5 days after encapsulation within the nematic gels ( Fig. 4c–e ), which indicates that the nematic gels are cytocompatible without compromising cell viability. Optical microscopy images of C2C12 collected over 2 days indicate that the density of the cells increases to form cell colonies in the gel matrix ( Supplementary Fig. S5a ), as opposed to growing as a monolayer on tissue-culture plastics (2D) ( Supplementary Fig. S5c ). This result demonstrates that the cells can proliferate in the 3D gel systems and, thus, the gels effectively offer a 3D culture environment to C2C12 cells. To confirm interactions between the cells and the gel matrices, we have performed cell culture experiments with the gels containing 10 mol% of RGD (Arg-Gly-Asp)-based rod amphiphile 3 . As shown in Supplementary Figure S6 , the cells express legs or filopodia, indicative of attachment of the cells to the nanofibre surfaces. Notably, we found that the encapsulated cells are released when the gels are cooled to temperatures below the sol–gel transition temperature ( Supplementary Figs S7 and S8 ). The ability of the gels to encapsulate and release cells that remain viable provides the potential for ex vivo cellular scaffolds. 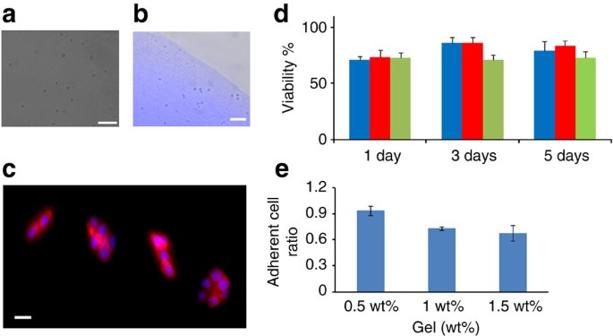Figure 4: Encapsulation of myoblast cells in nanofibre gels. (a) Optical image of encapsulated C2C12 cells in the nanofibre gel. (b) Differential interference contrast and blue fluorescence images for the cultured C2C12 cells were obtained at the same position. The blue region represents the nanofibre in imageb. (c) Fluorescent image of a stained cell after release from the gel. Red (actin) and blue (nucleus) fluorescence signals show that the cell was healthy. (d) The viability test using the water-soluble tetrazolium salt (WST) method of C2C12 cells grown in nanofibre gels (1 wt% (blue), 1.5 wt% (red) and 2 wt% (green)) for 5 days. (e) Calculated ratio of adherent cells to encapsulated cells using the CCK-8 assay solution after the cell release from various gel concentrations. The scale bars ina–care 100, 100, and 20 μm, respectively. The error bars indmean the standard deviations from four replicate experiments. The error bars inemean the standard deviations of the calculated adherent cell ratio from three replicate experiments. Figure 4: Encapsulation of myoblast cells in nanofibre gels. ( a ) Optical image of encapsulated C2C12 cells in the nanofibre gel. ( b ) Differential interference contrast and blue fluorescence images for the cultured C2C12 cells were obtained at the same position. The blue region represents the nanofibre in image b . ( c ) Fluorescent image of a stained cell after release from the gel. Red (actin) and blue (nucleus) fluorescence signals show that the cell was healthy. ( d ) The viability test using the water-soluble tetrazolium salt (WST) method of C2C12 cells grown in nanofibre gels (1 wt% (blue), 1.5 wt% (red) and 2 wt% (green)) for 5 days. ( e ) Calculated ratio of adherent cells to encapsulated cells using the CCK-8 assay solution after the cell release from various gel concentrations. The scale bars in a–c are 100, 100, and 20 μm, respectively. The error bars in d mean the standard deviations from four replicate experiments. The error bars in e mean the standard deviations of the calculated adherent cell ratio from three replicate experiments. Full size image We have been able to construct thermo-responsive nematic gels through the self-assembly of water-soluble nanofibres with a nematic substructure. The nematic alignment of the aromatic segments imparts a high fluorescence to the nanofibres because of J-aggregates within the core of the nanofibres. These fluoresent nematic gels spontaneously transform into a transparent solution upon cooling. The sol–gel transition allows for the encapsulation and growth of myoblast cells inside the 3D networks under physiological conditions. Consequently, the gels encapsulated C2C12 cells, which remained viable and were able to proliferate in a 3D environment, and subsequent cooling triggers the release of the encapsulated cells through a sol–gel transition. Liquid-crystal gels containing cells may be aligned along the fibre direction under appropriate conditions to yield macroscopically aligned monodomains for directional cell growth [11] , [39] . In this regard, we anticipate that our anisotropic gels will provide new opportunities for the construction of artificial extracellular matrices. Phase diagram The phase diagram of the aqueous solution of 2 was plotted by the tube inversion method using a water bath that can control temperature with a precision of ±0.05 °C. To ensure equilibrium, 20 min of equilibration time was allowed for each temperature. The gel formation was confirmed by the failure of the gel mixture to flow after the glass vial was inverted. Furthermore, the thermoreversibility of the gelation was confirmed by repeated heating and cooling cycles, which led to gel and liquid phases, respectively. Dynamic light scattering spectroscopy Dynamic light scattering measurements were performed using a He–Ne laser operated at 632.8 nm. The scattering was maintained at 90 °C during the entire experiment, and the temperature was maintained at 25 °C The hydrophobic diameter ( D H ) was determined from the autocorrelation functions by the time-interval method of photon correlation and the CONTIN methods using the software provided by the manufacturer. To avoid contamination by dust, all the solutions were filtered through a 0.45-μm membrane filter. TEM experiment For the study of the self-assembled structures of 1 and 2 in solution, a drop of solution of amphiphilic molecules was placed on a carbon-coated copper grid, and the solution was allowed to evaporate under ambient conditions. The samples were stained by depositing a drop of uranyl acetate onto the surface of the sample-loaded grid. The dried specimen was observed using a JEOL-JEM 2100 instrument operated at 120 kV. The data were analysed using the Digital Micrograph software package. Rheology We measured the rheological properties of the gels using a TA Instruments ARES-LS controlled strain rheometer with a cone-and-plate geometry at an angle of 0.396 rad and with a diameter of 25 mm. Dynamic frequency sweep measurements of 2 (3 wt%) were performed at 30 °C to monitor the G ′ (storage) and G ″ (loss) moduli at 3% strain and between frequencies of 0.1 and 100 rad s −1 to quantify the equilibrium behaviour. The sol–gel transformation, via temperature step changes, of 2 was monitored by dynamic time-sweep experiments performed at temperatures between 10 and 30 °C These time-sweep experiments were conducted at a frequency of 1 rad s −1 and 3% strain. When the temperature was increased from 10 to 30 °C, the gel was allowed to equilibrate for 1 h before the measurements were taken. In the cooling steps (30 to 10 °C), a longer time was allowed (~2 h) because of hysteresis in the disassembly of the gels. Cell culture in gels C2C12 cells were collected using trypsin–EDTA and were, then counted and resuspended in the complete medium (DMEM with 10% FBS). The cell suspension was mixed with nanofibre solutions at a final cell concentration of (5×10 4 cells per ml). A volume of 60 μl per well of the cell suspensions in nanofibres was allocated in 96-well plates, and the plates were maintained at 37 °C for 5 min to form a gel. DMEM with 10% FBS (20 μl) was added to each well, and the plates were maintained at 37 °C with 5% CO 2 . To observe cell morphology and growth, we used microscopy (X10; Axiovert 200M, Carl Zeiss). We obtained the images of the C2C12 cells in the nanofibres immediately after seeding, as well as images of cells at 1 and 2 days after seeding. Cell viability assay The C2C12 cells viability in the nanofibres was investigated using the Trypan blue assay and the EZ-Cytox Cell viability assay kit (water-soluble tetrazolium salt method). Trypan blue assay: At 1, 3 and 5 days after seeding the cells (1×10 4 cells per ml), three different concentrations of nanofibre gels (1, 1.5, 2 wt%) were changed to the solution state and C2C12 cells were collected on ice. The suspension of the cells in the nanofibre went down at 1,300 r.p.m., for 3 min and at 15 °C. The cells were then resuspended in a serum-free complete medium. The cell suspension was mixed with 0.4% Trypan blue (Sigma) and incubated for 3 min at room temperature. A drop of the Trypan blue/cell mixture was placed on a haematocytometer. Finally, we counted the unstained (viable) and stained (non-viable) cells separately in the haematocytometer. EZ-Cytox assay (dehydrogenase assay): At 1, 3 and 5 days after seeding the cells (1×10 4 cells per ml), the WST reagent solution (10 μl) was added to each well of a 96-well microplate that contained 100 μl of cells in the nanofibres at various gel concentrations (1, 1.5 and 2 wt%) under control conditions (96 wells for cell culture). The plate was then incubated for 3 h at 37 °C. The absorbance was measured at 450 nm using a microplate reader. At the same time, nanofibres without cells were incubated for 1, 3 and 5 days to obtain the background signal. As a result, we were able to calculate the final value: (total signal−background signal=original signal→(original signal/control signal)×100=viability%). How to cite this article : Huang, Z. et al . Responsive nematic gels from the self-assembly of aqueous nanofibres. Nat. Commun. 2:459 doi: 10.1038/ncomms1465 (2011).